Reconfigurable microfluidic hanging drop network for multi-tissue interaction and analysis Integration of multiple three-dimensional microtissues into microfluidic networks enables new insights in how different organs or tissues of an organism interact. Here, we present a platform that extends the hanging-drop technology, used for multi-cellular spheroid formation, to multifunctional complex microfluidic networks. Engineered as completely open, ‘hanging’ microfluidic system at the bottom of a substrate, the platform features high flexibility in microtissue arrangements and interconnections, while fabrication is simple and operation robust. Multiple spheroids of different cell types are formed in parallel on the same platform; the different tissues are then connected in physiological order for multi-tissue experiments through reconfiguration of the fluidic network. Liquid flow is precisely controlled through the hanging drops, which enable nutrient supply, substance dosage and inter-organ metabolic communication. The possibility to perform parallelized microtissue formation on the same chip that is subsequently used for complex multi-tissue experiments renders the developed platform a promising technology for ‘body-on-a-chip’-related research. Studying and understanding how living systems work depends to a large extent on the availability of suitable carefully engineered model systems, which should faithfully reproduce the biological system of interest. In vitro cell-based models constitute important test systems, as they allow for acquiring large data sets upon exposure to a broad variety of controlled stimuli and environmental changes. A wealth of highly automated analysis methods and tools is available for such in vitro studies. An important technological advancement was the introduction of microfabricated devices, which, in contrast to conventional culture dishes, allow for precisely manipulating cells at the micro- or nanometre scale and for handling of minute liquid volumes, so that microenvironments became highly controllable [1] , [2] , [3] . Over the last years, however, it became apparent that two-dimensional (2D) cell assemblies, grown on a flat substrate, have severe limitations in mimicking behaviour observed in the three-dimensional (3D) in vivo environment as morphological and biochemical features are different in 2D (refs 4 , 5 , 6 ). For mammalian tissues, cell-to-cell interactions and the presence of the extracellular matrix, which contains important proteins, provides structural support and mediates cell-to-cell communication, are very important features. Even though it is possible to precisely control the culture conditions of, for example, liver cells in 2D, they lose pivotal functional characteristics within a few days, which similarly holds true for other adherent mammalian cell systems [7] . This loss of function in 2D motivates the strong current effort to develop three-dimensional tissue structures, as they have been proven to exhibit properties that more closely resemble those of a living organism [6] , [8] , [9] , [10] . In analogy to the 2D case, microfluidic systems can be used to better control culturing conditions and to render those as similar as possible to the in vivo situation. Important parameters in this context include tissue-to-medium ratios, fluid residence times and dynamic mechanical forces that occur [11] . A next logical step is the development of fluidically inter-connected networks of 3D tissue structures, potentially derived from different cell types, which paves the way to a new generation of model systems for complex multi-tissue studies with the aim to ultimately being able to mimic the behaviour of larger organ networks of the human body (‘body-on-a-chip’ research initiatives) [12] , [13] , [14] , [15] , [16] , [17] , [18] , [19] , [20] , [21] . Combining 3D cell culturing with microfluidic structures implies several challenges. Many of the available 3D tissue formation approaches, which, in most cases, are already rather complex [22] , [23] , have been developed apart from microtechnological advancements, and are difficult to integrate without losing the functionality of the 3D tissue. Alternatively, specific microstructures and fluidic protocols have been designed to assemble cells into 3D tissue directly in the microdevices [24] , [25] so as to create models of, for example, lung [26] or liver [27] , [28] . For all approaches, reproducibility is a prerequisite to yield comparable studies. The microfluidic device itself primarily has to provide an optimal environment and robust tissue culturing over several days. This includes tight control of media and gas exchange. Simple tissue production and loading as well as simple operation of the device for tissue maintenance are pivotal for obtaining a user-friendly system and to enable a scale-up for highly parallel studies. Optical accessibility and reliable tissue harvesting are required for continuous monitoring and end-point analysis of the tissues. Many of the currently available systems are complex and designed for specific organ models. Multi-cellular spheroids or spherical microtissues (MTs), as used here, are scaffold-free cell clusters, which can be made from many cell types and are proven to feature tissue-like phenotype and functionality [29] , [30] . Owing to their relatively simple formation in hanging drops, spherical MTs have been a popular choice as developmental models for several organs [31] , [32] , [33] , [34] , [35] , [36] , [37] , [38] . Recently, spheroids have also been formed and characterized inside microfluidic systems [25] , [39] , [40] , [41] or transferred to those after external MT formation [42] . A major challenge arises from the presence of solid surfaces, to which cells tend to adhere, which, in turn, compromises reliable spheroid formation and cultivation. Anti-adhesive coatings have to be used to counteract surface adhesion of cells or cellular ensembles. Here, we present a highly versatile analytical platform for forming multi-cellular spheroids and conducting experiments with them. Our approach advances the frequently used hanging drop method towards fluidically interconnected hanging drop networks. The concept of interconnecting hanging drops in an array format and the capability to reconfigure these connections offer the following unique features: (i) controllable and reproducible spheroid formation from different cell types in parallel on the same platform, (ii) subsequent functional liquid interconnection of spheroids through microfluidic networks, (iii) controlled, continuous nutrient supply for developmental studies, (iv) microfluidic dosage of defined substance concentrations to the spheroids and (v) continuous fluidic communication between different spheroid types to enable complex multi-organ models, or so-called ‘body-on-a-chip’ experimental set-ups. Microfluidic device concept The microfluidic system has been realized by generating micropatterns on the surface of a subsequently inverted PDMS substrate ( Fig. 1 and Supplementary Note 1 ). Rim structures delimit wetted areas and prevent the liquid from spreading over the whole surface. When liquid is applied through an inlet, it is drawn through the network by capillary forces along the rims. With increasing pressure, drops are formed below the circular areas, the size of which is defined by the lateral distance of the rims and the surface tension at the liquid–air interface at the bottom. By variation of the lateral expansion of the liquid on the substrate it is, therefore, possible to define drops, which are used as spheroid compartments and interconnecting channels of different cross-sections: completely open, complex microfluidic networks of hanging drops can be designed. 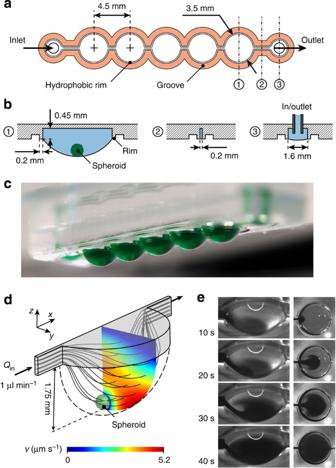Figure 1: Basic concept and flow characteristics of inter-connected hanging drops. (a) Layout showing five circular areas and channel structures defined by a rim, which prevents liquid from spreading over the whole surface of the device. (b) Cross-sections as indicated in (a) showing the inlet/outlet site with connected tubing, the 200-μm-wide channel, and the drop formed below the circular area with a base diameter of 3.5 mm. The liquid is restrained to the 450-μm-deep recess by the rim. Spheroids are located at the bottom of each drop. (c) Photograph of the device filled with food-dye-coloured de-ionized water showing equal-size drops (~14 μl per drop). (d) Numerically simulated streamlines and flow velocities of a perfused drop containing a 400-μm-diameter spheroid (applied flow rate is 1 μl min−1, hanging drop has maximal size and a height of 1.75 mm). The same flow rate is applied at the outlet. Grey areas indicate contact walls with no-slip condition (v=0 μm s−1). (e) Time-lapse photographs (10-s intervals) taken at an angle of ~45° from the side and from the top showing coloured liquid entering the drop (white semicircles are light reflections from the spherical drop surface). Figure 1: Basic concept and flow characteristics of inter-connected hanging drops. ( a ) Layout showing five circular areas and channel structures defined by a rim, which prevents liquid from spreading over the whole surface of the device. ( b ) Cross-sections as indicated in ( a ) showing the inlet/outlet site with connected tubing, the 200-μm-wide channel, and the drop formed below the circular area with a base diameter of 3.5 mm. The liquid is restrained to the 450-μm-deep recess by the rim. Spheroids are located at the bottom of each drop. ( c ) Photograph of the device filled with food-dye-coloured de-ionized water showing equal-size drops (~14 μl per drop). ( d ) Numerically simulated streamlines and flow velocities of a perfused drop containing a 400-μm-diameter spheroid (applied flow rate is 1 μl min −1 , hanging drop has maximal size and a height of 1.75 mm). The same flow rate is applied at the outlet. Grey areas indicate contact walls with no-slip condition ( v =0 μm s −1 ). ( e ) Time-lapse photographs (10-s intervals) taken at an angle of ~45° from the side and from the top showing coloured liquid entering the drop (white semicircles are light reflections from the spherical drop surface). Full size image Open conduits have previously been used to construct autonomous capillary systems [43] , [44] . The idea of inverting the substrates and including circular areas for drop formation within a network of fluidic channels has not been reported to date and offers completely new perspectives in association with multi-cellular spheroid cultures. The approach described here does not feature any solid surface to which cells could adhere at the bottom of the tissue compartments (hanging drops) or throughout the microfluidic network. The bottom surface is the liquid–air interface, which is key to preserving 3D tissue integrity and functionality in the hanging drops and preventing undesired cell adhesion in the microfluidic channels. The completely open system allows for optimal gas exchange during incubation (for example, oxygen and CO 2 ) and obviates any bubble formation, a frequent and severe problem in other systems during long-term perfusion. The liquid phase is accessible at every point in the network for sampling or harvesting of analytes or markers, cells and tissue structures. Cells and tissues can be imaged with high-resolution microscopy from the bottom. As channels are open at the bottom, the fluid dynamics, flow profiles and fluidic boundary conditions are different from those in closed microfluidic channels. Maximal flow velocities appear at the liquid–air interface and not—as it is common for a pressure-driven flow—in the centre of the channel ( Supplementary Note 2 ). This has the advantage that debris or unwanted single cells in the channels are easily washed away. The hanging drops do not have a fixed volume, because the bottom boundary—the liquid–air interface—behaves like a flexible membrane and deforms in response to variations in the liquid pressure in the fluidic network. Further, the flow conditions in the inverted compartments or hanging drops are different from those in conventional compartments in microfluidic systems (for details, see below). Owing to the availability of tissue compartments and connections, the approach described here allows for parallel spheroid formation and subsequent experimentation with the spheroids under conditions of continuous perfusion and media exchange. Moreover, metabolic inter-tissue communication can be established through microfluidic ducts, and specific signalling substances can be dosed while preserving functional interconnections. These novel features will be laid out and validated in the following sections of the article. Basic layout The basic layout consists of drops with 3.5 mm base diameter (in accordance with 384-well formats), interconnected through 0.2-mm-wide and 1-mm-long channels (pitch: 4.5 mm). Fig. 1a–c show a simple five-drop-row configuration. The dimensions have been optimized with regard to cell loading, drop and network stability, and perfusion characteristics ( Supplementary Note 2 ). A central feature is that the interconnected drops inherently exhibit the same size and volume, due to pressure equilibration as a result of the surface tension of the curved liquid–air interface (Young–Laplace equation: Δ p =2 γ / r ; Fig. 1c ): as a drop with fixed base diameter grows in volume, its radius decreases and reaches its minimal value, which is equivalent to the maximal internal pressure, at a hemispherical shape (here r =1.75 mm). Connected drops of different sizes are therefore exchanging liquid between each other until their radii are equal ( Supplementary Note 2 ). This feature is central for an equal distribution of cells over all drops during liquid loading and subsequent spheroid formation. Further, the hanging drop constitutes a natural well for the spheroid, which prevents the spheroids being washed away already at low flow velocities in the microfluidic network. The stable spheroid location simplifies long-term time-lapse imaging by using automated microscopes. The drops can be serially perfused by applying liquid flow to the inlet and outlet through the use of tubing connected from the top (back side of the microfluidic structure, see Supplementary Note 2 for time-lapse images). The laminar flow profile and the absence of the no-slip condition at the bottom drop–air interface of the liquid network causes spheroids, located at the bottom of the drop, being exposed to the highest flow speed in the drop ( Fig. 1d ). This ensures efficient media exchange ( Fig. 1e ). Maximal shear stress on the surface of a 400-μm-diameter spheroid at an applied flow rate of 10 μl min −1 and a drop height of 0.5 mm is 1.2 mPa, which is two orders of magnitude lower than values that have been reported as the maximal shear stress that, for example, hepatocytes can tolerate [45] ( Supplementary Fig. 1 ). Network stability The stability of such an open drop network is mainly determined by two factors: the drop radii and the fluidic resistances of the inter-connecting channels. The system can fail, when one of the drops is exceeding the volume of a hemisphere. Tilting of the microdevice causes hydrostatic pressure differences between drops, which induce flow. Smaller drops can withstand higher pressures until drip-off (for example, a drop with a base diameter of 3.5 mm can hold a water column of 8.5 mm in height). High channel resistances limit the flow. The dimensions of the microfluidic elements constitute, therefore, a trade-off between stability and flow requirements. The dimensions used here allow for convenient handling, as, for example, lateral microscope stage movements up to 25 mm s −1 , as well as quick tilting of the chip and even rapid flipping (<0.5 s)—so that the drops point upwards—are possible (please refer to Supplementary Note 2 for more details). A custom device mount was used for long-term measurements. Parallel spheroid formation The approach exhibits very large design flexibility for creation of complex, interconnected hanging-drop networks. This is demonstrated by implementing well-known microfluidic elements—after having taken into account that one channel wall is missing—for the parallel formation of spheroids under different conditions on the same chip. A four-by-four hanging-drop array was connected to a continuous-flow gradient generator [46] producing four different concentrations of a target compound of 0, 33, 67 and 100% of the original concentration by making use of integrated flow splitting and mixing structures ( Fig. 2a,b ). The four concentrations were fed in parallel to the four rows of drops. The equal flow rates in all four rows under a laminar flow regime yielded a constant concentration within the drops of the same row. Concentrated phosphate-buffered saline (10 × PBS), for example, has been diluted through the gradient mixer, and the resulting conductivity values have been compared with those obtained by manual, external dilution to identical concentrations: within experimental error, the values are the same. Moreover, there are only small variations between the values obtained from the four drops within the same row (s.d. <3%; Fig. 2c ). 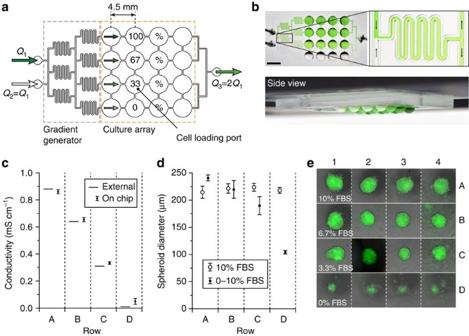Figure 2: Parallel spheroid formation. (a) Layout of the hanging microfluidic network consisting of a four-by-four array of drops with a diameter of 3.5 mm and a pitch of 4.5 mm. The array is fed in parallel with liquid that is diluted row-wise into four concentrations using a preceding gradient generator with two inlets, where equal flow rates are applied. The array has a single outlet, where liquid is withdrawn with twice the inlet flow rate and a single port for initial cell loading. (b) Photographs of the device from the top with a close-up view of the laminar flow conditions in the gradient generator and from the side. Food-dye is used to illustrate the working principle (scale bar, 5 mm). (c) Comparison of conductivities of 10 × PBS diluted manually and 10 × PBS diluted using the gradient generator. Samples were collected from each drop in each row (n=4, mean values, error bars are s.d.). (d) Diameters (n=4, means, error bars are s.d.) of HCT-116-derived spheroids, formed under static conditions in media containing 10% FBS and under conditions of varying FBS concentrations through the gradient mixer. (e) Micrograph overlay (bright-field and green fluorescence) of spheroids formed after 68 h in flow conditions with varying FBS concentrations (bright-field image at position C2 is compromised as a consequence of light scattering at the cell-loading port above the drop). Figure 2: Parallel spheroid formation. ( a ) Layout of the hanging microfluidic network consisting of a four-by-four array of drops with a diameter of 3.5 mm and a pitch of 4.5 mm. The array is fed in parallel with liquid that is diluted row-wise into four concentrations using a preceding gradient generator with two inlets, where equal flow rates are applied. The array has a single outlet, where liquid is withdrawn with twice the inlet flow rate and a single port for initial cell loading. ( b ) Photographs of the device from the top with a close-up view of the laminar flow conditions in the gradient generator and from the side. Food-dye is used to illustrate the working principle (scale bar, 5 mm). ( c ) Comparison of conductivities of 10 × PBS diluted manually and 10 × PBS diluted using the gradient generator. Samples were collected from each drop in each row ( n =4, mean values, error bars are s.d.). ( d ) Diameters ( n =4, means, error bars are s.d.) of HCT-116-derived spheroids, formed under static conditions in media containing 10% FBS and under conditions of varying FBS concentrations through the gradient mixer. ( e ) Micrograph overlay (bright-field and green fluorescence) of spheroids formed after 68 h in flow conditions with varying FBS concentrations (bright-field image at position C2 is compromised as a consequence of light scattering at the cell-loading port above the drop). Full size image Initial cell loading has been performed into an empty device. A defined liquid volume containing a defined number of cells has been applied with a single pipetting step through the cell-loading port on the top side of the device. A controlled pipetting flow and capillary effects distribute the liquid automatically through the whole network and lead to the formation of equal-size drops below the circular areas. At the same time, the cells have been homogeneously distributed over all 16 drop compartments. After pipette retraction, the cells located in each drop settle to the bottom and start to aggregate. In this way, 16 spheroids of equal size (220.2±7.9 μm, n =16) have been formed with only a single pipetting step ( Fig. 2d ). We could demonstrate scalability to up to 192 spheroids, formed in parallel with a single pipetting step in a 12-by-16 drop array (half a 384-well plate format). The s.d. in the spheroid diameter was <7% ( Supplementary Fig. 2 ). An applied continuous medium flow exposing the cells during aggregation to different concentrations of fetal bovine serum (FBS) in parallel (0, 3.3, 6.7 and the normally used 10%) resulted in significant differences in spheroid formation. Whereas FBS concentrations higher than 3.3% only affected the final spheroid sizes (more FBS led to larger spheroids), the absence of FBS (0%) prevented spheroid formation ( Fig. 2d,e ): the cells did not really aggregate. Harvesting of cells after culturing Recovery of 3D tissue from microfluidic culture devices is critical for subsequent analysis. Whereas this step may be challenging for closed systems, the open format of our device renders this procedure extremely simple. Spheroids can be removed directly from the bottom of the drop using a pipette aspirating a volume of 2–3 μl. A parallel spheroid transfer can be achieved by bringing all drops simultaneously into contact with a flat plate or with the wells of 384-well plate, similar to methods presented by Cavnar et al . [47] We easily could recover all spheroids from 16–24 drops without any loss of viability. Array reconfiguration In the previous section, we described how the arraying of hanging drops enables reproducible, parallel spheroid formation and continuous perfusion of the formed MTs. For more complex multi-tissue studies, the fluidic inter-connection of spheroids of different sizes and/or spheroids derived from different cell types is desirable. We implemented this option with on-demand reconfiguration of the connection between the hanging drops by using capillary valving [43] ( Fig. 3a ). A smaller group of hanging drops in the network, for example, one column in the four-by-four array, has been initially isolated from the rest and filled through the respective cell-loading port with a specific cell solution to form equal spheroids ( Fig. 3b ). The cell-loading port is located sideways from the array and is accessible from the top. The same step has then been repeated for each of the other columns with different cell solutions through the respective loading ports. Capillary valves between the columns prevent the liquid from flowing into the neighbouring columns during cell loading. The valves consist of a sharp widening of the channel, which creates a pressure barrier, which the entering liquid is not able to overcome. Once cells were settled, a small volume of medium was introduced through the connection ports (located on the other side of the array of Fig. 3a ) to break the capillary valves and enable liquid transfer between the columns, and to connect all the columns into a four-by-four drop array. Introducing identical volumes in each column results in equal drop sizes and a negligible media crossover. Subsequently, the array was connected to the adjacent perfusion elements including the gradient generator and the outlet channels. Spheroids derived from different cell types in the different columns can now interact across columns upon starting perfusion, when liquid flows horizontally from one drop to the next. This option substantially increases device versatility and offers the potential to perform complex experiments with multiple spheroids derived from different cell types. In the present device design, four different tissue spheroids (four columns) located now in series in one row can be exposed to a certain compound concentration, and four concentrations can be applied in parallel (four rows). 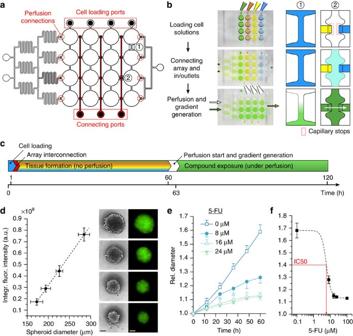Figure 3: Array reconfiguration. (a) Layout of the four-by-four drop array, showing the added features for array reconfiguration (marked in red). Cell-loading ports have been shifted to the top of the array; connecting channels have been added between the columns; valves have been introduced to connect the perfusion channels (red circles). (b) Three handling steps are required during an experiment (close-up views show key areas): First, four different cell solutions are applied at the loading ports. Second, the isolated columns are connected via liquid introduced through the connecting ports so that the horizontal perfusion channels are open and useable. Third, perfusion is started and generates a gradient flow through the array (highest concentration in bottom row). (c) Time protocol of the substance exposure experiment. (d) Linear correlation (R2=0.9988) of diameter and fluorescence measurements of formed spheroids by using bright-field and fluorescence micrographs acquired 60 h after seeding (n=4, mean values, error bars are s.d.; scale bars, 100 μm). (e) 5-FU-dependent growth of the spheroids over 60 h: diameter increase relative to the initial diameter (n=4, mean values, error bars are s.d.). (f) Dose response curve including the results of experiments, performed with higher 5-FU concentrations (0–100 μM,n⩾4, mean values, error bars are s.d., fitted Hill-Function,R2=0.996). Figure 3: Array reconfiguration. ( a ) Layout of the four-by-four drop array, showing the added features for array reconfiguration (marked in red). Cell-loading ports have been shifted to the top of the array; connecting channels have been added between the columns; valves have been introduced to connect the perfusion channels (red circles). ( b ) Three handling steps are required during an experiment (close-up views show key areas): First, four different cell solutions are applied at the loading ports. Second, the isolated columns are connected via liquid introduced through the connecting ports so that the horizontal perfusion channels are open and useable. Third, perfusion is started and generates a gradient flow through the array (highest concentration in bottom row). ( c ) Time protocol of the substance exposure experiment. ( d ) Linear correlation ( R 2 =0.9988) of diameter and fluorescence measurements of formed spheroids by using bright-field and fluorescence micrographs acquired 60 h after seeding ( n =4, mean values, error bars are s.d. ; scale bars, 100 μm). ( e ) 5-FU-dependent growth of the spheroids over 60 h: diameter increase relative to the initial diameter ( n =4, mean values, error bars are s.d.). ( f ) Dose response curve including the results of experiments, performed with higher 5-FU concentrations (0–100 μM, n ⩾ 4, mean values, error bars are s.d., fitted Hill-Function, R 2 =0.996). Full size image Open-loop parallel substance exposure The reconfiguration of a hanging drop array is demonstrated by an open-loop continuous-flow exposure of differently sized HCT-116 eGFP-derived spheroids to fluorouracil (5-FU), a cytostatic substance used for the treatment of cancer. The substance has been chosen as its effects on cells or tissues are well characterized. Cell solutions of different cellular concentrations (15,000, 25,000, 40,000 and 70,000 cells per ml) have been sequentially loaded into the four array-columns via the corresponding ports ( Fig. 3c ). Once the cells have settled, medium has been applied through the connection ports to interlink the array and through inlets and outlets to fill the perfusion channels. During the next 60 h, spheroids of different sizes have formed in dependence on the initial cell concentrations in the drops ( Fig. 3d and Supplementary Movie 1 ). MT size variations in the columns are below 10% (rel. s.d. ), and they are linearly correlated to the overall GFP fluorescence intensity per spheroid. After spheroid formation has been completed, continuous perfusion is started. Medium with 24 μM of 5-FU is infused through one of the two inlet ports, whereas medium without the substance is infused through the second port at the same flow rate (1 μl min −1 ). The 24-μM 5-FU solution is diluted to concentrations of 0, 8, 16 and 24 μM by the gradient generator before reaching the drop array. At the outlet, liquid is withdrawn at twice the flow rate (–2 μl min −1 ) of the inlet in order to keep the drops at a constant size. The substance gradient over the full array has been slowly built up within 3 h and then been maintained for the rest of the experiment (60 h) through continuous flow. 5-FU has a significant impact on the growth of the HCT-116 spheroids of all sizes ( Fig. 3e ). Control spheroids continue to grow and increase in diameter, relative to the initial diameter, as a result of cell proliferation (+68±6%). The growth of spheroids exposed to 8 μM of 5-FU is significantly reduced (+28±3%). Higher concentrations result in the expected cytostatic effect of 5-FU (+15±2%). The apparent IC50 value of 5.6 μM compares well to that reported in literature ( Fig. 3f ) [48] . Parallel closed-loop bio-activation In a next step we used a similar configuration to validate the device suitability for parallelized multi-tissue experiments ( Fig. 4a ). We realized a hepatic pro-drug activation experiment, which differs from other recent work [17] , in the used pro-drugs, cell types, device structure (cells in chambers with hydrogels) and microfluidic approach. The array consisted of four columns and six rows. Again, each column hosted the same type of spheroids. Here, the first three columns have been used to form spheroids derived from freshly isolated rat liver cells (rLiMT; ~1800 cells per drop and tissue, respectively). In the fourth column, HCT-116 eGFP cancer spheroids have been formed (250 cells per drop). After cell seeding and array connection, no cellular cross-talk between column 3 and 4 has initially been observed ( Fig. 5a ), that is, no fluorescent HCT-116 cells have been detected in the neighbouring liver cell column ( Fig. 5b ). Spheroids have been formed in 4–5 days with diameter variations of <8% ( n =12) in the case of rLiMTs and <10% ( n =36) for HCT-116 MTs ( Supplementary Movie 2 ). Subsequently, the array has been horizontally perfused in a closed-loop format along the rows by using an external peristaltic pump for up to 8 days ( Fig. 4b ). Three different concentrations of cyclophosphamide (CP; 0.0, 0.1 and 1.0 mM) have been added to the medium. Each concentration has been applied to two neighbouring rows by making use of the laminar flow regime. CP is a well-known prodrug-type anticancer agent effective against a broad range of human cancers, but only after hepatic activation ( Fig. 4c ) [49] . Briefly, CP is converted to 4-hydroxycyclophosphamide (CP-OH) by the hepatic cytochrome P450 (CYP) isozymes. The tautomer of CP-OH, aldophosphamide, circulates and passively enters other cells, where it undergoes a spontaneous (non-enzymatic) elimination reaction to yield phosphoramide mustard, which, in turn, crosslinks DNA strands. 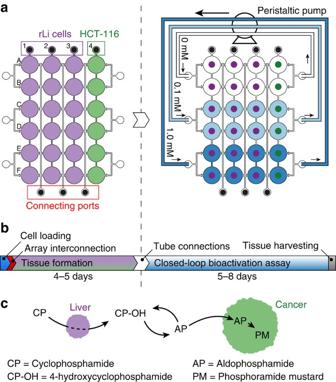Figure 4: Experimental layout for bio-activation experiments. (a) Layout of the device indicating the cell types in the respective drop columns: Columns 1–3 have been loaded with hepatocytes, column 4 contains HCT-116 cancer cells. After reconfiguration, rows are horizontally perfused in a closed-loop format; pairs of channels receive the same CP concentrations. Laminar flow prevents lateral crosstalk. (b) Time protocol of the bio-activation experiment. (c) Simplified pathway of the CP activation. Figure 4: Experimental layout for bio-activation experiments. ( a ) Layout of the device indicating the cell types in the respective drop columns: Columns 1–3 have been loaded with hepatocytes, column 4 contains HCT-116 cancer cells. After reconfiguration, rows are horizontally perfused in a closed-loop format; pairs of channels receive the same CP concentrations. Laminar flow prevents lateral crosstalk. ( b ) Time protocol of the bio-activation experiment. ( c ) Simplified pathway of the CP activation. 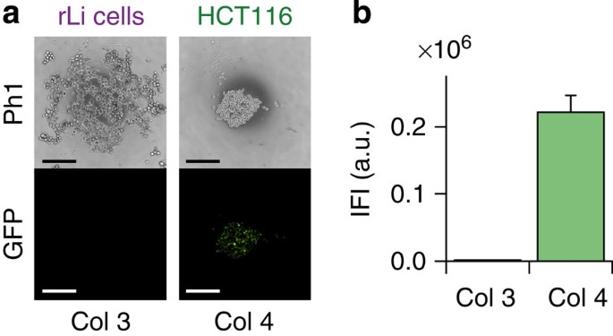Figure 5: Loading crossover. (a) Phase contrast (Ph1) and fluorescence (GFP) micrographs of drop A3 and A4 inFig. 4a(scale bars, 100 μm), and (b) integrated fluorescence intensities of all drops in columns 3 and 4 just after loading and inter-connection of the array (n=6, mean values, error bars are s.d.). No crossover is detectable, which would imply cells travelling from column 4 to column 3. Full size image Figure 5: Loading crossover. ( a ) Phase contrast (Ph1) and fluorescence (GFP) micrographs of drop A3 and A4 in Fig. 4a (scale bars, 100 μm), and ( b ) integrated fluorescence intensities of all drops in columns 3 and 4 just after loading and inter-connection of the array ( n =6, mean values, error bars are s.d.). No crossover is detectable, which would imply cells travelling from column 4 to column 3. Full size image We were able to reproduce the bio-transformation described in Fig. 4c , by loading liver and cancer tissues in the same device and by applying continuous perfusion across the different tissue types while dosing two different CP concentrations as well as no CP for control on the same single device. Time-lapse imaging over the full duration of the experiment shows the different slopes of relative fluorescence intensity increase of the spheroids in dependence of three conditions: 0.0, 0.1 and 1.0 mM CP in the circulating medium ( Fig. 6a , Supplementary Fig. 3 and Supplementary Movie 2 ). The final spheroid fluorescence intensities ( Fig. 6c ) and the relative spheroid sizes ( Fig. 6d ) show significant differences and demonstrate the impact of metabolized CP on tumour growth. After 132 h of continuous perfusion, HCT-116 spheroids were harvested and tested for ATP content ( Fig. 6e ). The results confirm the optical observation. As a control, HCT-116 spheroids were exposed to CP in absence of hepatocytes at the same flow conditions. No significant direct effect of CP on HCT-116 spheroids has been observed ( Fig. 6b ). 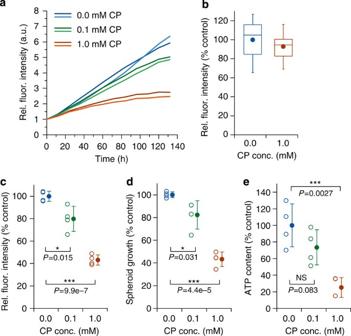Figure 6: Parallel bio-activation experiment. (a) Normalized fluorescence intensity curves over 132 h of one of the experiments showing inhibited growth in the presence of CP in the medium at different concentrations. Each experiment includes all three conditions (0.0, 0.1 and 1.0 mM CP) in duplicates. (b) Control experiment showing no measurable direct effect of CP on HCT-116 eGFP spheroids in the absence of liver tissue (n=10, box plot and mean). (c) End-point fluorescence intensities of HCT-116 eGFP spheroids after 132-hour, closed-loop perfusion (244 h total experiment time including 112 h of spheroid formation) relative to intensities after formation (n=4, mean values, error bars are s.d.). (d) Growth of HCT-116 eGFP spheroids after 132-hour, closed-loop perfusion (244 h total experiment time including 112 h of spheroid formation,n=4, mean values, error bars are s.d.). (e) ATP content of spheroids of each type of exposure (n=4, mean values, error bars are s.d.). Figure 6: Parallel bio-activation experiment. ( a ) Normalized fluorescence intensity curves over 132 h of one of the experiments showing inhibited growth in the presence of CP in the medium at different concentrations. Each experiment includes all three conditions (0.0, 0.1 and 1.0 mM CP) in duplicates. ( b ) Control experiment showing no measurable direct effect of CP on HCT-116 eGFP spheroids in the absence of liver tissue ( n =10, box plot and mean). ( c ) End-point fluorescence intensities of HCT-116 eGFP spheroids after 132-hour, closed-loop perfusion (244 h total experiment time including 112 h of spheroid formation) relative to intensities after formation ( n =4, mean values, error bars are s.d.). ( d ) Growth of HCT-116 eGFP spheroids after 132-hour, closed-loop perfusion (244 h total experiment time including 112 h of spheroid formation, n =4, mean values, error bars are s.d.). ( e ) ATP content of spheroids of each type of exposure ( n =4, mean values, error bars are s.d.). Full size image In parallel we conducted two similar bio-activation experiments in 96-well plates by using a protocol involving discrete pipetting steps to interchange medium between the wells. Three preformed primary rat liver MTs (rLiMT) were either cultured in separate wells or were pooled together in order to increase the cell-to-medium volume ratio. Total media volumes were chosen similar to those used in the microfluidic device. Media containing CP at concentrations of 0.1 and 1.0 mM and media without CP have been incubated with the rLiMTs for 2 days (first small effects on tumour growth started to occur after 2 days in the perfusion microfluidic systems) and have then been transferred to wells containing a single HCT-116 eGFP spheroid. The media have been transferred via single pipetting steps in a circular way every 2 days (see Supplementary Figs 4a and 5a for details). For both experimental layouts and for both CP concentrations we did not observe any significantly reduced tumour spheroid growth over a time of 6 and 8 days, respectively, in culture in comparison to control experiments without CP. No direct effects of CP on HCT-116 eGFP spheroids as well as minor effects on rLiMTs were observed ( Supplementary Figs 4 and 5 ). Whereas the control experiments for microfluidic devices and for the pipetting transfer produce similar results, there is a clear difference in the case of the bio-activation experiments. These findings illustrate the importance of continuous liquid and metabolite transfer between the different tissues or tissue compartments. In isolated spheroid configurations such transfer could only be achieved with frequent discrete media exchanges. Suitable transfer timings and long-enough incubation times to obtain the desired metabolic compounds are, however, difficult to estimate and optimize. Further, the comparably large well volumes of conventional set-ups may entail a too-large dilution of the active metabolites. Increasing the cell-to-medium volume ratio by co-culturing spheroids in the same droplet or well leads to uncontrolled tissue fusion in short time; too-large agglomerates also develop necrotic cores ( Supplementary Fig. 5e ). The above findings demonstrate that the use of isolated hanging drops or well formats with an already labour-intensive pipetting protocol cannot reproduce the results obtained with continuous media exchange, as has been exemplified for a set-up including only two different tissue types. For experimental scenarios requiring more than two different tissue types, pipetting approaches are no more an option, as the respective protocols become very complex, whereas microfluidic networks offer viable solutions. Hanging drops have been used since decades for the production of spherical MTs. They rely on the liquid–air interface at the bottom of the drop where cells settle without any risk of adhesion. Aggregation of a variety of cell types into 3D tissue structures in hanging drops has been demonstrated. The simplicity of production and handling together with the better representation of in vivo -like cell behaviour—as compared with 2D single-layer cell cultures—renders spheroids very attractive as developmental tissue models for multiple biosystems and organisms. A major drawback of the hanging-drop method is the fact that spheroids are isolated in their respective drops and that media exchange and the metabolic communication with other tissue types has to be carried out through multiple discrete pipetting steps. Linking hanging drops into a microfluidic network is, therefore, a missing key feature in currently available hanging drop methods and substantially expands the experimental options for the use of spherical MTs. First, MT production can be further scaled up and simplified due to the option of parallelization and due to substantial reduction in pipetting steps. Second, controlled perfusion is possible and allows for nutrient supply and substance dosage; additionally, continuous circulation and transfer of substances, such as metabolic compounds, between different drops is enabled, which can be pivotal, as has been observed in bio-activation studies. Third, and most importantly, MT production, cultivation and exposure experiments can be combined in the very same platform. These advantages can even be better exploited by integration of simple valving, as has been demonstrated. MTs derived from different cell types can be produced in the same microdevice, and subsequent liquid transfer (including marker or signalling molecules) between the different tissue types becomes possible. Parallel multi-tissue experiments with programmable perfusion protocols are made available. This is particularly attractive, as models of different organs can be simultaneously produced, which makes the platform a universal tool for multi-organ arrangements. Compared with other 3D tissue models, spheroids do not need any solid supports, hydrogels, scaffolds or matrices to obtain a 3D arrangement. The integration of such solid supports or scaffolds into a microfluidic environment could be laborious and may pose challenges with regard to reproducibility of conditions and experiments. The idea of inverting a substrate and using a completely open microfluidic structure is key to our approach. The resulting devices offer all functions described above and can be fabricated with simple chip-processing steps; the device handling is convenient and the experimental set-up is robust. On the fabrication side, only the patterning of a single substrate surface is required, which renders our approach compatible with other technologies, such as injection moulding, so that the devices can be made disposable. The rim structure, which defines the lateral dimensions of the drops and channels, can be geometrically varied with great flexibility in order to fabricate a broad range of microfluidic networks for diverse experimental configurations. No additional cover for channel closure is needed. No additional materials or active parts have to be integrated, which entails short fabrication times and low costs. Further, the open system is directly accessible to optical imaging and liquid sampling, as well as to MT harvesting for further analysis. Gas exchange is ensured, and undesired bubble formation is inexistent. Another important issue in using microfluidics is a bubble-free initial filling of the channel structures, especially for multiply branched networks. While phase guides, microfabricated rims to guide liquids for a controlled filling of large reservoirs and to prevent bubble trapping in corners, can be used in closed systems [50] , the entrapment of bubbles is rarely occurring in the open systems presented here. Further, the surface tension of the drops actively transports the liquid through the system until complete equilibration throughout the whole system. The drops and their surface tension characteristics act as small, integrated pumps, so that large and complex systems can be reliably filled through a single inlet. Finally, off-chip fluidic connections are kept to a minimum and can simply be plugged into the system from the top. All liquid handling can be performed with standard pipettes or syringe pumps. The different examples in this paper provide evidence of the large potential of the described approach for a new analytical platform. Regular drop arrays as well as more complex functional drop networks have been presented, and commonly used microfluidic features, such as laminar flow, serial and parallel channel arrangements with channel resistance adjustment, or gradient generators have been demonstrated. Spherical MTs were reproducibly formed in parallel on-chip in variable sizes and from different cell types, encompassing common cell lines as well as primary cells. Reconfiguration of drop arrays enabled crossed-flow configurations with column-wise formation of spheroids from different cell types and subsequent row-wise medium perfusion while applying different compound concentrations. Experiments ran stable without bubble formation for >10 days, a time span, which included spheroid formation and compound testing. For future applications, the central advantages of the presented approach include the possibility to establish continuous inter-drop (or inter-tissue) fluidic communication and perfusion, and a large flexibility in designing the respective microfluidic networks to enable a broad variety of experiments, which cannot be done in isolated hanging drops. Medium exchange, which has to be carried out in discrete steps via pipetting, can become very complex and labour-intensive in classical hanging-drop arrays. Pipetting and discrete medium changes do, however, not occur in the body, where there are gradual changes mediated by liquid flow or transport of specific molecules. Moreover, the transfer of very low concentrations of metabolites occurs continuously within a body with comparably short transport times. Therefore, we believe that interconnected hanging drop networks more closely resemble the conditions in a living organ or organism and have the potential to generate more representative results. Finally, the presented technology enables the realization of more complex MT systems, featuring a larger number of different tissue types (>2), and enables to simulate a continuous physiological liquid exchange—similar to that between the organs of a body—for all those tissue types. In summary, we demonstrated that complex 3D cell-based assay protocols can be executed on a single microfluidic platform that features high usability and a multitude of functions, while handling complexity is kept at a minimum. We are confident that our platform can play an important role in gaining new systemic or holistic insights, for example, into human organ systems by using human-derived 3D spherical tissue models. Microfluidic device fabrication Microfluidic structures have been created through casting poly(dimethylsiloxane) (PDMS, Sylgard 184, Dow Corning Corp., USA) using a microfabricated SU-8 mould. Two layers of SU-8 (Microchem Corp., USA) have been spin-coated consecutively onto a 4-inch silicon wafer to achieve the desired thicknesses of h 1 =200 μm and h 2 =250 μm. UV exposure through the respective transparency mask to initiate crosslinking has been executed after the soft bake of each layer. Development of all unexposed and, therefore, not crosslinked SU-8 was done at the end of the photolithographic process. The obtained SU-8 master constitutes the negative of the final microfluidic structure in PDMS. Before PDMS casting, the moulds were coated with trichloro(1 H ,1 H ,2 H ,2 H -perfluorooctyl)silane (Sigma-Aldrich, Switzerland) in a vapour silanization process in order to reduce adhesion. PDMS was poured onto the SU-8 structure at a thickness of ~3 mm, cured for 2 h at 80 °C and cut to desired device sizes. Fluidic access holes were punched at the inlet and outlet sites. For better stability and planarity, the PDMS layer was bonded after oxygen plasma activation to a microscopy slide (25 mm × 75 mm, 1 mm thick) featuring drilled liquid access holes. The detailed protocol is available in Supplementary Note 1 . Cell culture Fluorescent human colorectal carcinoma cells (HCT-116 eGFP, Sirion Biotech, Germany) were cultured in RPMI 1640 growth medium (Chemie Brunschwig AG, Switzerland), supplemented with 10% fetal FBS (Sigma-Aldrich), 100 IU ml −1 penicillin, 100 μg ml −1 streptomycin (P/S, Chemie Brunschwig AG) and 0.3 μg ml −1 Puromycin. The culture was maintained in a humidified incubator at 37 °C in 5% CO 2 (Heracell 150i, Thermo Scientific, USA). Cell culturing was carried out according to routine protocols. Briefly, cells were pre-cultured until reaching 80% confluence. Before starting an experiment, the cells were cultured to confluence, and then digested with 0.25% trypsin/EDTA solution (in growth medium, Life Technologies, Switzerland). The cell suspension was centrifuged, and the cell pellet was washed twice with PBS (Life Technologies). The cells were re-suspended in fresh growth medium. Cell density was measured using a haemocytometer and adjusted according to the requirements of the experiment. Primary cell isolates from rat liver were received from InSphero AG, Switzerland, and directly used after isolation. Gradient characterization The microfluidic gradient generator has been validated using 10-fold concentrated PBS (10 × , Sigma-Aldrich), introduced at a flow rate Q 1 of 25 μl min −1 through one inlet, and de-ionized water, introduced at the same flow rate Q 2 =25 μl min −1 through the second inlet. The withdrawal flow rate at the outlet was set to Q 3=–50 μl min −1 . Ten microlitres were sampled directly from every drop using a conventional pipette. Between sampling, a volume of at least 300 μl (twice the chip volume) was pumped through the chip to restore the gradient. Samples were diluted to a concentration of 1:200 in de-ionized water in order to adjust liquid volume and conductivity for the conductivity measurements (sensor linear range 0.1–10 mS cm −1 , JUMO GmbH & Co. KG, Germany). For comparison, we prepared the same dilution series manually. Microfluidic cell culture Before the experiments, the microfluidic chips were rinsed with acetone and isopropanol and dried using an air gun. The wettability of PDMS was increased by applying oxygen plasma. In order to ensure drop stability, the patterned surface was covered with a thin PDMS layer featuring openings only at the drop sites. This procedure resulted in a localized surface modification that keeps the top area of the rim around the drops and along the channels hydrophobic and prevents liquid overflow. For all experiments the microdevices were inserted into a custom-made chip holder, placed in a covered one-well culture dish. Humidifier cotton pads soaked with PBS were placed at the bottom of the culture dish in order to reduce water evaporation from the drops. The chip holder fixes the microscope slide with the PDMS microstructures facing down. Cell loading was performed using conventional 10-μl and 100-μl pipettes. Defined volumes of media with the corresponding cell concentrations were pumped through the cell-loading ports into the empty device at a flow rate of ~10 μl s −1 . For microdevices with the option for reconfiguration, media (3–5 μl) were applied 10–15 min after cell loading through the respective ports. Perfusion channels were filled from inlets and outlets with media. After complete loading, the microfluidic structures were inspected optically for correct filling. Initial target drop heights were in the range of 0.8–1.0 mm. For continuous perfusion, PTFE tubing (ID 0.5 mm, OD 1.0 mm, Bohlender GmbH, Germany) was connected to the respective inlets and outlets. In the case of spheroid aggregation without perfusion, tubing was only connected after spheroid formation was completed. Flow rates were controlled using precision syringe pumps. For closed-loop experiments, peristaltic pumps (IPC and IPC-N, IDEX Health & Science GmbH, Switzerland) with prefilled tubing were used. Parallel spheroid formation HCT-116 eGFP cell solution (160 μl) featuring a concentration of 40,000 cells per ml (RPMI 1640 media, +10% FBS, +1% P/S) was loaded in a single pipette-step into the central inlet port ( Fig. 2a ) to create all 16 drops and to fill all channels including those of the gradient generator. The rather high flow rate ensures equal distribution of ~375 cells per drop (10 μl used for perfusion channels). After 60–90 min, cells settled to the bottom of each drop. The static spheroid formation has been performed without any media exchange. For the perfusion experiment with varying FBS concentrations, RPMI 1640 medium including 10% FBS and 1% P/S was introduced through one inlet at a flow rate of Q 1 =1 μl min −1 and RPMI 1640 medium (+1% P/S) without FBS through the second inlet at Q 2 =1 μl min −1 . The withdrawal rate at the outlet was set to Q 3=–2 μl min −1 . Time-lapse images (phase contrast and green fluorescence) were acquired at 15-min intervals. Open-loop parallel drug exposure Tissues of different sizes were produced by introducing media with different cell concentrations into each column. Each column was filled with 50 μl of medium containing 15,000, 25,000, 40,000 and 70,000 cells per ml, which resulted in ideally 190, 310, 500 and 880 cells per drop. The cells were allowed to pre-settle during 5 min. Then medium was introduced through the connection ports (~3 μl). The drop connection events are visible to the eye. Finally, medium was introduced through the two inlets (~10 μl each) and the outlet (~5 μl), thereby connecting the gradient generator and perfusion channels. Inlet ports were left open during the overall duration of the experiment. The array reconfiguration has to be performed shortly after cell loading as PDMS re-establishes its native hydrophobic surface, which renders subsequent capillary filling impossible. Spheroids were formed under static conditions for 60 h. Bright-field and fluorescence images were taken every 30 min. Once spheroids were formed, tubing was connected to inlets and outlet. Medium only and medium containing 24 μM (or 100 μM respectively) of 5-FU (from 24/100 mM stock solution in 100% DMSO, Sigma-Aldrich, resulting in a final concentration of 0.1% DMSO in the medium) were infused through the inlets at 1 μl min −1 using precision syringe pumps (neMESYS, Cetoni GmbH, Germany). A flow rate of –2 μl min −1 was applied at the outlet. Experiments with food colour showed that the gradient was established within 2–3 h, corresponding to a total liquid turnover of twice the chip volume. These flow conditions remained unchanged for the next 60 h. Time-lapse imaging of every drop was performed as before. Closed-loop bio-activation Cells were loaded directly after chip preparation. Primary cells isolated from the rat liver were diluted in re-aggregation medium (HHRM, InSphero AG, Switzerland) to a cell concentration of 160,000 cells per ml. The comparably high cell concentration was necessary, because primary cells do not proliferate. Cell suspension (65 μl) was loaded into each of the three columns resulting in ideally 1,730 cells per drop. HCT-116 eGFP cells were loaded into the 4th column at a concentration of 40,000 cells per ml (RPMI 1640, +10% FBS, +1% P/S). RPMI medium was used to inter-connect the array and perfusion channels. After spheroid formation was completed, peristaltic tubing (120 μl volume) was connected to the respective inlets and outlets for closed-loop perfusion. The peristaltic tubing was prefilled with maintenance medium (HHMM, InSphero AG) containing CP (Sigma-Aldrich) at concentrations, which yielded the respective target concentrations of 0.1 and 1.0 mM upon dilution with the medium already present in the drop rows. The total liquid volume of two four-drop rows including tubing was 270 μl. Control experiments with only HCT-116 eGFP were performed at the same experimental conditions. Compensating evaporation Even though humidifier cotton pads and a controlled microenvironment with a microscope stage top incubator were used, we could not completely eliminate a reduction of the drop heights over time due to liquid evaporation from the open system. The evaporation rates varied with the respective microdevice and experimental set-up and were determined experimentally. For static cultures and closed-loop perfusion set-ups, additional medium was added periodically by using a programmable syringe pump (Harvard Apparatus Pump11 Elite, Hugo Sachs, Germany) connected to one of the inlets. For static cultures in the four-by-four array, medium was added at a rate of 1.3 μl h −1 (8 μl every 6 h at 2 μl min −1 ). For closed-loop cultures (four-by-six array), the evaporation rate was calculated to 3.5 μl h −1 and also compensated by liquid addition. In the case of the open-loop perfusion with the four-by-four array, the evaporation was compensated by pausing the liquid withdrawal every 6 h for 4 min (1.3 μl h −1 ). Spheroid culture Spheroids derived from HCT-116 eGFP cells were formed in the GravityPLUS plate following the protocol of the manufacturer (InSphero AG, Switzerland). RPMI 1640 media (40 μl; +10% FBS, +1% P/S) containing 250 cells was pipetted from the top into the funnel-like structure producing the hanging drop. After an incubation time of 4 days in a humidified CO 2 incubator at 37 °C (Heracell 150i, Thermo Scientific, USA), spheroids were formed and then transferred into a pre-wetted GravityTRAP plate (InSphero AG) for subsequent experiments. Well-plate bio-activation experiments The experiments included one pre-formed HCT-116 eGFP spheroid (see above) and three primary rat liver spheroids (rLiMT, 7 days after isolation, obtained from InSphero AG, Switzerland). rLiMTs were (i) either cultured in separate wells with 70 μl HHMM media or were (ii) pooled in a single well with 70 μl HHMM media of a GravityTRAP plate (InSphero AG). HCT-116 eGFP spheroids were cultured in separate wells with 70 μl of RPMI 1640 (+10% FBS, +1% P/S) medium. CP (Sigma-Aldrich) has been added to both media (HHMM and RPMI 1640) at concentrations of 0.0, 0.1 and 1.0 mM. Experiments were carried out in a humidified CO 2 incubator. Every 2 days media have been transferred between the wells in discrete pipetting steps as follows: (i) 20 μl of each well containing individual rLiMTs have been removed and transferred to the HCT-116 eGFP well, whereas 60 μl have been removed from the HCT-116 eGFP well, split into three 20-μl aliquots and transferred back to the rLiMT wells ( cf . Supplementary Fig. 4a ); (ii) 60 μl of medium have been exchanged between the well containing the three pooled rLiMTs and the single HCT-116 eGFP spheroid ( cf . Supplementary Fig. 5a ). Image acquisition Microfluidic cell culture experiments were performed on a NIKON Ti Eclipse inverted fluorescence microscope with a motorized xy-stage (NIKON, Switzerland), and a stage-top incubator to control temperature (37 °C), humidity (>95%) and CO 2 levels (5%) (Life imaging services, Switzerland). Bright-field (phase contrast) and fluorescence time-lapse images were acquired with × 10 extra-long working distance objective and a Hamamatsu ORCA Flash 4.0 camera at time intervals of 10–30 min using an automated stage positioning and software-based autofocusing (2 × 2 binning mode). The light source for bright-field images was a CoolLED pE-100 (CoolLED Ltd., Andover, UK) and for green fluorescence images a SPECTRA X light engine (Lumencor Inc., Beaverton, OR, USA; 470/24 nm excitation wavelength, 495 nm dichroic beam splitter, 525/50 nm emission filter). Spheroids in well plates have been analysed by using a Leica DFC 340FX CCD camera, mounted on an inverted microscope (Leica DMI6000, Leica, Switzerland). Only bright-field images were taken using the standard microscope configuration. Image analysis Time-lapse images were analysed using the ImageJ or the NIS Elements Advanced Research Analysis software (NIKON, Switzerland). Diameters were measured manually or calculated from bright-field images. For the latter, marks (>5) were manually placed on the border of the spheroids, which were used to fit a circle. Integrated GFP intensities were calculated after background subtraction. ATP assay HCT-116 eGFP MTs were collected after the CP bioactivation experiment, and the ATP content was evaluated using the CellTiter-Glo 3D Luminescent Cell Viability Assay (Promega, Switzerland) following the manufacturer’s protocol. ATP concentrations were compared against standard dilutions using a microplate reader (Infinite M200pro, TECAN, Switzerland). FEM modelling 3D computational fluid-dynamic simulations were performed with the COMSOL Multiphysics software version 3.5a using steady-state analysis in the incompressible Navier–Stokes module. Results were consolidated by varying the element size of the 3D mesh. Lateral symmetry was exploited to reduce the element number. The drop was assumed to be constant in size, and the MTs were assumed not to be displaced by drag force. The liquid–air interfaces were modelled using the ‘slip’ boundary condition, whereas the ‘no-slip’ condition was applied at the liquid–substrate interfaces. Inflow and outflow regions were extended in order to enable the development of a parabolic flow-profile. Statistical analysis All error bars are s.d.. If no error bars are indicated, the s.d. is smaller than the size of the symbol representing the mean in the graph. ‘ n ’ refers to the number of data points if not specified otherwise. Significance criteria rely on a one-tailed, two-sample unequal variance Student’s t -test using * P <0.05, ** P <0.01 and *** P <0.005. No samples were excluded. All experiments have been conducted with n ⩾ 4. In some cases multiple experiments were required to achieve n ⩾ 4. How to cite this article: Frey, O. et al . Reconfigurable microfluidic hanging drop network for multi-tissue interaction and analysis. Nat. Commun. 5:4250 doi: 10.1038/ncomms5250 (2014).